Coherent multidimensional optical spectra measured using incoherent light Four-wave mixing measurements can reveal spectral and dynamics information that is hidden in linear spectra by the interactions among light-absorbing molecules and with their environment. Coherent multidimensional optical spectroscopy is an important variant of four-wave mixing because it resolves a map of interactions and correlations between absorption bands. Previous coherent multidimensional optical spectroscopy measurements have used femtosecond pulses with great success, and it may seem that femtosecond pulses are necessary for such measurements. Here we present coherent two-dimensional electronic spectra measured using incoherent light. The spectra of model molecular systems using broadband spectrally incoherent light are similar but not identical to those expected from measurements using femtosecond pulses. Specifically, the spectra show particular sensitivity to long-lived intermediates such as photoisomers. The results will motivate the design of similar experiments in spectral ranges where femtosecond pulses are difficult to produce. Systems as diverse as atomic gases, molecules, proteins, polymers and semiconductor nanostructures have been studied using four-wave mixing spectroscopy [1] , [2] , [3] , [4] , [5] , [6] , [7] , [8] , [9] . The measurements have led to new insights into energy transfer, peptide secondary structure, many-body interactions and other phenomena. Four-wave mixing measurements exploit the third-order nonlinear optical response of the material under study. Variants such as transient absorption use sequences of short laser pulses—often femtoseconds in duration—to probe or coherently control dynamics directly in the time domain [10] , [11] ; other variants such as coherent anti-Stokes Raman scattering use continuous-wave (cw) laser excitation to probe spectral properties directly in the frequency domain [1] ; even other four-wave mixing measurements combine the two domains [12] , [13] . Coherent multidimensional optical spectroscopy is an important type of four-wave mixing measurement because it resolves correlations between excitation and emission frequencies of the signal as a function of a variable time delay [6] , [9] . The spectroscopic technique—analogous to multidimensional NMR spectroscopy [14] —has been performed in the infrared, visible and ultraviolet spectral regions [15] , [16] , [17] , [18] , [19] , [20] , [21] , [22] , [23] , [24] , [25] , [26] , [27] , [28] . In the visible region, the technique is often called two-dimensional electronic spectroscopy (2D ES), and it has been used to study important topics such as photosynthetic energy transfer [29] , [30] , [31] , [32] . As a consequence of how we think about timing using femtosecond laser pulses, coherent multidimensional optical spectroscopy seems to require coherent excitation. A first femtosecond excitation pulse ( E A ) interacts with the sample to induce coherent superpositions between the ground and excited states; these polarizations oscillate at optical frequencies. After a delay τ 1 , a second excitation pulse ( E B ) interacts to induce either populations of the ground or excited states or low-frequency coherent superpositions known as quantum beats inside the ground-state or excited-state manifolds. After a delay τ 2 , a third excitation pulse ( E C ) interacts to induce new coherent superpositions between the ground and excited states that oscillate at optical frequencies. These polarization oscillations lead to emission of a coherent signal field ( E sig ) during the third time period, τ 3 , in the phase-matched direction. Using a weak local-oscillator field ( E LO ) and a phase-stable interferometer, the influence of the amplitude and phase of each excitation field on the emitted signal field can be measured as a function of all three time intervals. The oscillations at optical frequencies during τ 1 and τ 3 are usually presented in the Fourier domain as a 2D spectrum. Dynamics are often displayed parametrically by presenting a 2D spectrum for each τ 2 value. On the basis of the description, short laser pulses do seem necessary to measure coherent 2D spectra because the phase of the coherence needs to be preserved during τ 1 and τ 3 . Indeed, to date, all coherent multidimensional optical spectra have been measured using coherent laser excitation [15] , [16] , [17] , [18] , [19] , [20] , [21] , [22] , [23] , [24] , [25] , [26] , [27] , [28] , [29] , [30] , [31] , [32] , [33] , [34] . The vast majority of measurements used femtosecond pulses and even small deviations from a perfectly linear spectral phase profile introduce artefacts [33] , [34] . Here we report coherent 2D optical spectra measured using quasi-cw incoherent light, I (4) 2D ES, where I (4) means four incoherent excitation fields. Using incoherent excitation in conjunction with time-domain interferometry, we observe that strong four-wave mixing signals can be generated in the phase-matched direction; that an LO field can be used to extract relative phase and amplitude information; and that coherent oscillations at optical frequencies can be measured and then Fourier transformed to produce 2D spectra. The 2D spectra contain similar but not identical information as 2D spectra measured using femtosecond pulses. The 2D measurements using incoherent light are extensions of one-dimensional (1D) four-wave mixing spectroscopy measurements using incoherent excitation, a field referred to as noisy-light spectroscopy [35] , [36] , [37] , [38] , [39] , [40] . The main feature of noisy-light spectroscopy is that the time resolution is given by the coherence time of the light, and not the temporal envelope. In principle the noisy beams can be cw, although in practice they are often pulsed on the order of hundreds of nanoseconds. This is still essentially cw relative to femtosecond and picosecond material dynamics. Measurement using time-integrated detection We used broadband-amplified spontaneous emission (ASE) and a four-beam interferometer to measure I (4) 2D ES using time-integrated detection; more details are presented in Methods. We chose to study the carbocyanine dye 1,1′-diethyl-2,2′-tricarbocyanine perchlorate (DTP) in butanol as a model system. One can gain significant intuition about I (4) 2D ES by reviewing how a Michelson interferometer can be used to measure a linear absorption spectrum. Both I (4) 2D ES and Fourier-transform linear absorption spectroscopy are coherent spectroscopy techniques that use spectrally incoherent light; both use multiple-beam interferometers; and both rely on time-correlation functions as part of the signal detection method. 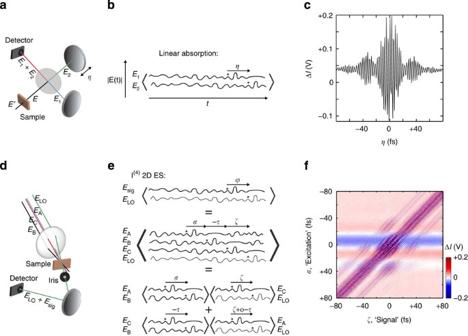Figure 1: Relationship between linear absorption spectroscopy and I(4)2D ES. (a) Optical apparatus for linear absorption spectroscopy uses a two-beam interferometer with interferometric delayηbetween armsE1andE2. (b) The wiggly lines represent the envelope of the electric field of noisy light as a function of time, and the * indicates a common relative time point in the otherwise identical noisy beams for ease of viewing. Brackets indicate the two-point time-correlation function intrinsic to intensity-level detection. (c) Measured 1D interferogram of DTP in butanol shows coherent oscillations at optical frequencies. (d) Optical apparatus for 2D spectroscopy uses a four-beam interferometer with interferometric delaysσ,τandζbetween armsEA,EB,ECandELO. We depict the time-integrated measurement; we used a spectrometer and CCD instead of a photodiode in the frequency-resolved measurements. (e) In I(4)2D ES, the detected time-correlation function betweenEsigandELOis recast as a four-point time-correlation function by considering the four-wave mixing process. The intractable four-point time-correlation function can then be broken down into products of two-point time-correlation functions. (f) Measured 2D interferogram of DTP in butanol forτ=0. Coherent oscillations at optical frequencies persist in all four quadrants. Figure 1 depicts the two measurements. We present theoretical analysis in Methods and in ref. 40 ; below we provide physical descriptions. Figure 1: Relationship between linear absorption spectroscopy and I (4) 2D ES. ( a ) Optical apparatus for linear absorption spectroscopy uses a two-beam interferometer with interferometric delay η between arms E 1 and E 2 . ( b ) The wiggly lines represent the envelope of the electric field of noisy light as a function of time, and the * indicates a common relative time point in the otherwise identical noisy beams for ease of viewing. Brackets indicate the two-point time-correlation function intrinsic to intensity-level detection. ( c ) Measured 1D interferogram of DTP in butanol shows coherent oscillations at optical frequencies. ( d ) Optical apparatus for 2D spectroscopy uses a four-beam interferometer with interferometric delays σ , τ and ζ between arms E A , E B , E C and E LO . We depict the time-integrated measurement; we used a spectrometer and CCD instead of a photodiode in the frequency-resolved measurements. ( e ) In I (4) 2D ES, the detected time-correlation function between E sig and E LO is recast as a four-point time-correlation function by considering the four-wave mixing process. The intractable four-point time-correlation function can then be broken down into products of two-point time-correlation functions. ( f ) Measured 2D interferogram of DTP in butanol for τ =0. Coherent oscillations at optical frequencies persist in all four quadrants. Full size image In linear absorption, coherent signals can be detected even when they are generated by incoherent sources. The incident field ( E ′) excites different molecules at different times, and it may seem that the total response—if measured as a superposition of induced signal fields—would average to zero. However, the detected signal arises because the field radiated by each molecule ( E sig , the free polarization decay) interferes destructively with the E ′ that produced it. This reduces the intensity of the transmitted field ( ) compared with the E ′, and it occurs because the amplitude and phase of E sig are intrinsically locked to E ′. In other words, the sample reduces the amplitude of certain frequencies. These reductions will be revealed by the time-correlation function operation central to the time-integrated detection method using a Michelson interferometer, as depicted in Fig. 1a . A beam splitter produces two copies of E so that the two arms, E 1 and E 2 , are identical stochastic functions of time except for a relative interferometric delay η . The two beams recombine and the sum is detected by a photodiode. Detection of the cross terms at the intensity level is a time-correlation function, . We depict this in Fig. 1b using wiggly lines to indicate the electric field amplitude as a function of the laboratory time variable t and angle brackets to indicate the time-correlation function. Individually, the electric fields depicted in Fig. 1b do not have obvious reference points for timing femtosecond processes because they are stochastic functions of time. We are able to extract meaningful information about the sample only by interferometric correlation. For each value of η , the background-subtracted voltage provides the amplitude and sign of the correlation. We recorded the voltage as a function of η , shown in Fig. 1c , to yield the signal for the model system. Coherent oscillations due to the electronic transitions of the sample—which occur at optical frequencies—are evident. One could create the sample absorption spectrum presented in Fig. 2a by processing the Fourier transforms of two scans, one with the sample (shown in Fig. 1c ) and the another without it (not shown). 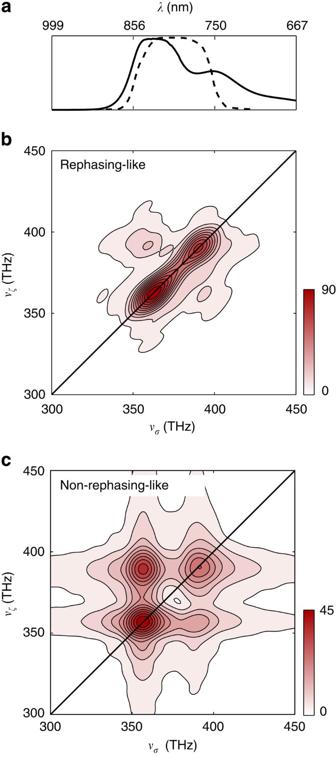Figure 2: I(4)2D ES from time-integrated data set. (a) The linear absorption spectrum of DTP in butanol and the noisy-light excitation spectrum are displayed in the solid and dashed lines, respectively. (b) The ‘rephasing-like’ spectrum atτ=0 has two prominent diagonal peaks and two weak cross peaks. The reduced antidiagonal linewidth is discussed in the text. The horizontal and vertical axes correspond to excitation and emission frequencies, respectively. (c) The ‘non-rephasing-like’ spectrum atτ=0 shows prominent diagonal and cross peaks. The cross peaks indicate coupling between the two transitions. The upper cross peak has a larger amplitude than the lower cross peak, indicating the presence of a photoisomer; see Discussion for more description about this feature of I(4)2D ES. Figure 2: I (4) 2D ES from time-integrated data set. ( a ) The linear absorption spectrum of DTP in butanol and the noisy-light excitation spectrum are displayed in the solid and dashed lines, respectively. ( b ) The ‘rephasing-like’ spectrum at τ =0 has two prominent diagonal peaks and two weak cross peaks. The reduced antidiagonal linewidth is discussed in the text. The horizontal and vertical axes correspond to excitation and emission frequencies, respectively. ( c ) The ‘non-rephasing-like’ spectrum at τ =0 shows prominent diagonal and cross peaks. The cross peaks indicate coupling between the two transitions. The upper cross peak has a larger amplitude than the lower cross peak, indicating the presence of a photoisomer; see Discussion for more description about this feature of I (4) 2D ES. Full size image A similar principle as above helps us to explain how the third-order nonlinear response is produced and detected with noisy light. As the third-order signal field is a stochastic function of time, we need to lock its amplitude and phase to the E ′s. We accomplish this by producing multiple copies of the E ′ using a phase mask in a four-beam interferometer [41] , Fig. 1d . The four fields are identical except for relative interferometric delays σ , τ , and ζ . In the BOX geometry, three of these fields, E A , E B and E C , excite the molecules to produce a third-order signal field, E sig , in the phase-matched direction collinear with the local-oscillator field E LO . A photodiode detects the heterodyned signal. The measured intensity is proportional to the correlation between E LO and E sig , , see Fig. 1e , where we have introduced a fourth interferometric delay variable, φ , between E LO and E sig . This is done as a matter of explanatory convenience; the value of φ is determined in part by the experimentally controlled interferometric delays but can in principle depend on the material response as well. For each setting of φ , the (stochastic) E LO acts as a temporal anchor on the laboratory time frame t against which the (stochastic) E sig is correlated, similar to the Michelson interferometer. As the fields that produce E sig are identical to E LO , an interferometric scan over variable φ yields a 1D spectrum but is insufficient for producing a 2D spectrum. To make progress, we use knowledge of the four-wave mixing process to recast the time-correlation function between E LO and E sig as the four-point time-correlation function depicted in Fig. 1e , . The four-point time-correlation function contains the three interferometric delay variables under complete experimental control but is intractable. We employ the standard assumption of circular complex Gaussian statistics [42] to obtain , where the two-point time-correlation functions are easier to evaluate and interpret. This expansion is depicted in Fig. 1e . The three interferometric variables remain in the two-point time-correlation functions, and a scan over any of the interferometric variables will lead to signal oscillations in a manner similar to the above example of linear absorption spectroscopy. Oscillations due to the electronic transitions of the sample at optical frequencies during σ and ζ are shown in the measured data presented in Fig. 1f . A more rigorous description of I (4) 2D ES relies on the formalism for nonlinear optical responses convolved with the details of how the optical fields are correlated. In standard descriptions of nonlinear optical spectroscopy, the signal field is expanded perturbatively in the light–matter interaction. For the third-order nonlinearity used here, there are multiple pathways for signal generation often called Liouville pathways [2] . The key difference between femtosecond and noisy-light 2D measurements is that in the former, the interferometric delays correspond directly to the interaction-time variables in the Liouville pathways. In the latter, the interferometric delays correspond only to the delay between identical time points along noisy electric fields. Any arbitrary point on the time profile of the noisy field can conceptually serve as such an ‘anchor point’, an idea closely related to the ‘fingerprint region’ concept in the noisy-light literature [35] , [36] , [37] , [38] , [39] , [40] . The asterisks in the schematics of the noisy-light fields shown in Fig. 1b,e mark an arbitrarily chosen anchor point. The parameters η , σ , τ and ζ give experimental control over the delay between corresponding anchor points. The time at which any given field can act upon the sample is not under experimental control because of the quasi-cw nature of the noisy light. Therefore, all possible time orderings for the field–matter interactions have a role in producing the four-wave mixing signal. The non-trivial correspondence between the interaction-time variables in the Liouville pathways and the interferometric delays can be depicted and understood using a formalism cast in terms of factorized time-correlation diagrams. See refs 39 , 40 for a detailed description of this formalism. As depicted in Fig. 1e , two of the interferometric delay variables will respect the interaction times in a manner similar to femtosecond methods. However, the third will not; see Methods for more details. We acquired the data presented in Fig. 1f by scanning σ and ζ from −80 to +80 fs with a step size of 0.8 fs at τ =0. Although almost all femtosecond 2D spectroscopy measurements use frequency-resolved detection, we performed this first measurement using time-integrated detection to be consistent with the I (4) 2D ES theory [40] and nearly all 1D noisy-light measurements, including refs 35 , 36 , 37 , 38 , 39 . We highlight the signal as function of ζ with σ =0 in Fig. 1c . Using the projection-slice theorem and assuming negligible contribution from excited-state absorption pathways, this trace is identical to a linear absorption measurement. The measured signal shows oscillations at optical frequencies corresponding to the electronic transitions as the interferometric delay ζ is scanned. The measured 2D data show that the intensity-level signal oscillates at optical frequencies in all four quadrants, that beats between at least two frequencies are apparent, and the signal persists at long σ and ζ times along the line σ =− ζ . These observations are all consistent with the previous theoretical work [40] . The persistent signals along σ =− ζ are in large part because of terms that account for the symmetry of the two non-conjugate fields, E A and E C ; the terms originate from the second pair-correlator product depicted in Fig. 1e . In previous work [40] , these were dubbed β-type unrestricted terms, and from the Bloch model it followed that the signals persist along σ =− ζ for the excited-state lifetime. Here we stopped the scan at 80 fs. The consequence of this truncation appears in the resulting spectrum as apodization of the antidiagonal linewidth. I (4) 2D spectra from the time-integrated data set We produced the I (4) 2D ES by Fourier transformation of the zero-padded data from two quadrants of the time–time data set. We did not make subcycle timing adjustments to each beam; thus, the so-called global phase was not corrected [41] , [43] . Instead, we present magnitude I (4) 2D ES displayed on linear colour scales. In femtosecond 2D ES, the direct relation between the interferometric delay setting and the interaction times of the Liouville pathways means that the rephasing (non-rephasing) pathways only generate signal as part of the rephasing (non-rephasing) pulse-timing sequence. In I (4) 2D ES, because the light is always on, any Liouville pathway (rephasing, non-rephasing and two-quantum) can potentially contribute at any interferometric delay setting. In other words, although the ranges of the interferometric delays mimic certain types of femtosecond 2D ES measurements, the Liouville pathways are not restricted in the same manner. We therefore label Fig. 2b,c the ‘rephasing-like’ and ‘non-rephasing-like’ spectra, respectively. The rephasing-like spectrum originated from the quadrant of the time–time data set and the non-rephasing-like spectrum originated from the quadrant. We present the linear absorption spectrum of DTP in butanol and the spectrum of the incident light source in the solid and dashed lines, respectively, in Fig. 2a . The two lowest-frequency transitions of the sample are centred at 826 nm (363 THz) and 750 nm (400 THz). Measurements and I (4) 2D ES using frequency-resolved detection Theoretical analysis, raw data, and scan and data treatment details are presented in Supplementary Notes 1–4 , Supplementary Tables S1–S4 and Supplementary Figs S1–S15 . Briefly, we used a spectrometer and charge-coupled device (CCD) camera to detect the heterodyne frequency-resolved signal using a noisy-light version of spectral interferometry. This allowed rapid data acquisition but required a new theoretical analysis; ref. 40 and Supplementary Note 1 are relevant only to time-integrated detection. In Supplementary Note 2 and Supplementary Tables S1–S4 , we present analysis and results, respectively, for frequency-resolved detection of noisy-light four-wave mixing signals. The analysis in Supplementary Note 3 and simulation results in Supplementary Figs S4 and S5 indicate that spectral interferometry methods similar to those used in femtosecond 2D ES should work, and indeed this is confirmed by experiments. Acquisition of a 2D spectrum at one τ value required about 2 min using frequency-resolved detection, whereas time-integrated detection required about 10 h. Using this frequency-resolved detection method, we studied two complementary model systems to explore further the photoisomer signatures: DTP in butanol and anhydro-11-(4-ethoxycarbonyl-1-piperazinyl)-10,12-ethylene-3,3,3′,3′-tetramethyl-1,1′-di(3-sulfopropyl)-4,5;4′,5′-dibenzoindotricarbocyanine hydroxide (IR144) in a 1:4 mixture of methanol and ethylene glycol. In Fig. 3 , we present the I (4) 2D ES of DTP in butanol at τ =100 fs at three different excitation energies. The lowest-excitation energy of 6 nJ per pulse is equivalent to the energy used in femtosecond 2D ES measurements. The spectra were ‘phased’ using the projection-slice theorem in the same manner used in femtosecond 2D ES measurements (see Supplementary Note 4 ). The spectra in Fig. 3 are total correlation spectra—the sum of the rephasing-like and non-rephasing-like components—which eliminate phase-twisted lineshapes in the same manner as femtosecond 2D ES measurements. The spectra show similar asymmetry as Fig. 2c ; the above-diagonal cross peak is significantly brighter than the below-diagonal cross peak. 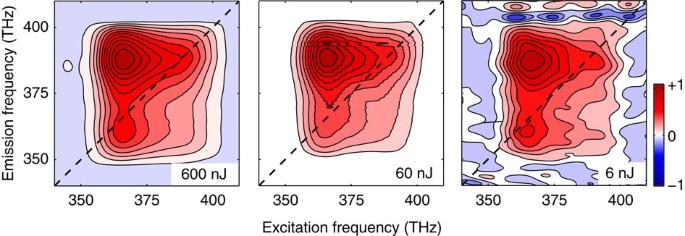Figure 3: I(4)2D ES of DTP from frequency-resolved data sets. Each spectrum is the real part of the total correlation spectrum atτ=100 fs. The three measurements differ only in excitation fluence. As in the time-integrated detection results presented inFig. 2c, the above-diagonal cross peak is significantly brighter than the below-diagonal cross peak. Figure 3: I (4) 2D ES of DTP from frequency-resolved data sets. Each spectrum is the real part of the total correlation spectrum at τ =100 fs. The three measurements differ only in excitation fluence. As in the time-integrated detection results presented in Fig. 2c , the above-diagonal cross peak is significantly brighter than the below-diagonal cross peak. Full size image In Fig. 4 , we present measurements on IR144, a prototypical laser dye used in countless femtosecond spectroscopy measurements, for example, an initial report of femtosecond 2D ES [15] . We show the linear absorption spectrum and the noisy-light excitation spectrum in Fig. 4a . In Fig. 4b,c , we present I (4) 2D ES of IR144 measured at two different pulse energies. The two I (4) 2D ES differ in the amount of noise because of scatter. These spectra are total correlation spectra at τ =200 fs. In IR144, the below-diagonal cross peak is significantly brighter than the above-diagonal cross peak, and this was independent of excitation spectrum (see Supplementary Figs S9 and S10 ). 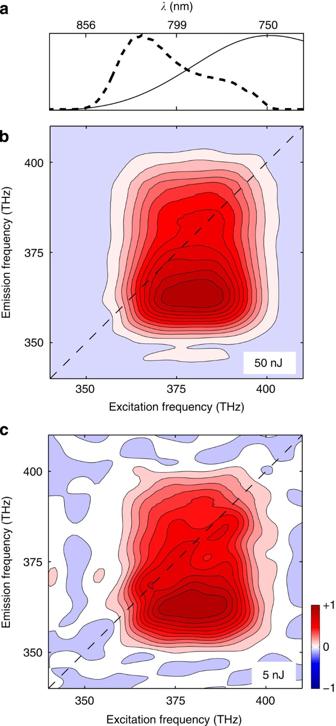Figure 4: I(4)2D ES of IR144 from frequency-resolved data sets. (a) The linear absorption spectrum of IR144 in a 1:4 mixture of methanol and ethylene glycol and the noisy-light excitation spectrum are displayed in the solid and dashed lines, respectively. The spectra inbandcare the real part of the total correlation spectra atτ=200 fs. The below-diagonal cross peak is brighter than the above-diagonal cross peak. Figure 4: I (4) 2D ES of IR144 from frequency-resolved data sets. ( a ) The linear absorption spectrum of IR144 in a 1:4 mixture of methanol and ethylene glycol and the noisy-light excitation spectrum are displayed in the solid and dashed lines, respectively. The spectra in b and c are the real part of the total correlation spectra at τ =200 fs. The below-diagonal cross peak is brighter than the above-diagonal cross peak. Full size image Previous noisy-light measurements involved homodyned 1D four-wave mixing, but the most straightforward implementation of coherent 2D spectroscopy requires relative amplitude and phase information not measureable using homodyne detection. Recent theoretical work predicted that 2D spectra could be measured using incoherent light with heterodyne detection of a four-wave mixing signal [40] . The first result reported here exactly follows the time-integrated formulation described in ref. 40 . We furthermore extend the previous theoretical work to frequency-resolved detection, which significantly decreases data acquisition time. The measurements confirm that coherent 2D optical spectroscopy measurements can be performed with spectrally incoherent excitation. The results mean that 2D spectroscopy requires a broadband light source but not necessarily femtosecond laser pulses, which are spectrally coherent. We describe the technique from the perspective of linear absorption spectroscopy—a measurement that can be performed with light of any spectral coherence—rather than from the perspective of femtosecond 2D spectroscopy. This qualitative description is useful, although it does not capture all of the important details underpinning the experiment. We envision one advantage of using incoherent excitation to measure 2D spectra is that users are not constrained by the costs and challenges associated with producing and controlling femtosecond laser pulses, which can be particularly difficult in the ultraviolet spectral region, for example. Another possible application is at even shorter wavelengths, such as 2D spectroscopy using X-rays [44] , where it is also challenging to produce broadband transform-limited pulses. A third possible application is to apply the method described here directly to probe photochemical species such as photoisomers or triplet states, whose signatures can be weak in femtosecond 2D ES but strong in I (4) 2D ES. The spectra shown in Fig. 2 reflect characteristic features of the absorption spectrum of DTP. Diagonal peaks appear at 358 and 391 THz; these frequencies correspond to the two transitions observed in the linear absorption spectrum (slightly truncated by the excitation bandwidth and the measurement resolution). The lower-frequency peak is the electronic S 0 → S 1 transition, whereas the higher-frequency peak is a bright vibronic transition. Cross peaks between the two transitions are evident, particularly in the non-rephasing-like spectrum ( Fig. 2c ). The cross peaks indicate that the two transitions share a common ground state; microscopically, the two transitions involve the same molecular orbitals (indeed, the same electronic states). Cross peaks are one of the most important features in 2D spectra because they directly reveal couplings, which are ultimately the source of electronic and vibrational dynamics. In this measurement, the cross peaks are due to strong coupling of a 37-THz (1,220 cm −1 ) vibrational mode to the main electronic transition [45] . Such modes have also been shown to lead to cross peaks in femtosecond 2D ES studies of similar molecules [22] , [41] , [46] , [47] . Our equipment cannot produce femtosecond pulses with more than about 10 nm of bandwidth at 800 nm, and therefore we were unfortunately not able to perform the equivalent 2D measurement using femtosecond pulses. The diagonal peaks dominate the rephasing-like spectrum in Fig. 2b . The antidiagonal linewidths of the diagonal peaks are smaller than the diagonal linewidths, but this does not indicate inhomogeneous broadening as would be expected from femtosecond 2D spectroscopy. This is a significant difference between the femtosecond and noisy-light methods. In femtosecond rephasing measurements, the ratio of the antidiagonal linewidth to the diagonal linewidth contains information about the relative contributions from homogeneous and inhomogeneous line broadening. In the noisy-light spectrum performed here at τ =0, following the Bloch model [40] , the antidiagonal linewidth yields the excited-state lifetime because the group of terms that directly probe the lifetime decay accumulate signal strength by integrating over dephasing times in a constant manner during this experimental scanning scheme. Ideally, σ and ζ should be scanned to times beyond the excited-state lifetime, which is not practical in this case because the excited-state lifetime of DTP is about 30 ps (ref. 48 ), whereas the maximum scan range of the instrument is about 0.5 ps. The value of the excited-state lifetime is also important to determine the strength of certain subsets of signal pathways, see Methods. Although modest compared with many laser dyes, the 30-ps timescale is sufficiently longer than the optical dephasing time of about 20 fs such that we expect steady-state terms (those of unrestricted topology in ref. 40 ) to be at least 1,000 times stronger than the dynamic terms (those of singly and doubly restricted topology in ref. 40 ); the timescale is also short enough compared with the excitation pulse duration (about 150 ns, see Supplementary Fig. S6 ) to ensure that the cw approximation is valid [40] . The signals from β-type unrestricted terms could be eliminated to reveal the conventional inhomogeneous broadening information by either setting τ to a value larger than the dephasing time or to use two uncorrelated light sources, one producing E A and E B and the other producing E C and E LO . The cross peak amplitudes in Figs. 2c and 3 represent a singular aspect of I (4) 2D ES. Spectroscopists often use cross peaks in femtosecond 2D ES to probe the dynamics of energy transfer; one expects that the below-diagonal cross peak—where the excitation energy is greater than the emission energy—should increase in amplitude as a function of waiting time as higher-lying excited states decay to the lower-energy state via intramolecular relaxation. Yet in the measurements of DTP, the above-diagonal cross peak is brighter than the below-diagonal cross peak. On the other hand, the below-diagonal cross peak is brighter than the above-diagonal cross peak in the measurement of IR144. The imbalance in both measurements persists at all values of τ , in multiple solvents and under a broad range of pulse spectrum excitation conditions, see Supplementary Figs S9 and S10 . A reasonable explanation for the difference in the cross peak amplitudes of the two samples is that DTP photoisomerizes but IR144 does not. Indeed, the end groups used in the infrared (IR) family of laser dyes were developed to be bulky enough to prevent photoisomerization [45] . In many carbocyanine dyes including DTP, photoexcitation causes one or more bonds in the polymethine chain to isomerize. The photoproduct is blue shifted relative to the primary excitation of the all- trans ground state [45] , [49] . Although the lifetime of the excited singlet state is on the order of picoseconds in DTP, photoisomers in carbocyanines can live for microseconds or even milliseconds at room temperature in solution [45] . Probing photoisomerization in femtosecond spectroscopy typically requires significant data analysis of weak but long-lived features [50] , [51] . In contrast, in I (4) 2D ES the powerful unrestricted terms integrate over the long lifetime, and thus lead to strong spectral features, indicating the presence of photochemical species. Thus, one big difference between I (4) 2D ES and femtosecond 2D ES is that the amplitude of features in I (4) 2D ES are proportional to the lifetime of species. This can be used to amplify spectral signatures of photochemical products or intermediates. The linear absorption spectra show that the vibronic shoulder of IR144 is not as clearly resolved as the vibronic shoulder of DTP, and therefore the cross peaks in the I (4) 2D ES of IR144 are less clearly resolved than the cross peaks in the I (4) 2D ES of DTP. Nevertheless, the overall rectangular shape—consistent with numerous femtosecond 2D ES measurements of similar carbocyanine molecules where vibronic splittings do not exceed absorption linewidths [22] , [25] , [28] , [41] , [46] , [47] —of the IR144 2D spectra indicate that both diagonal and cross peaks are present. The results in Figs 3 and 4 show that the signals are robust over a wide range of excitation energies. The peak irradiance used in many femtosecond experiments is about 10 10 W cm −2 . The lowest-excitation conditions in this work—5 nJ per pulse delivered in about 150 ns in an area <0.02 mm 2 —correspond to a peak irradiance of about 10 2 W cm −2 . Sunlight delivers about 0.1 W cm −2 . Thus, the lowest-excitation conditions correspond to about 1,000 suns, an excitation level achieved in high-concentration photovoltaic cells [52] . As described in Methods, even lower-excitation energies should generate detectable four-wave mixing signals. We envison that these results will clarify and refocus the debate surrounding the interpretation of coherent oscillations in 2D ES recorded using femtosecond laser pulses. Several groups studied the interpretation of femtosecond 2D ES measurements of photosynthetic proteins and what those measurement reveal about the natural conditions for photosynthesis [53] , [54] , [55] , [56] by focusing on the distinction between spectrally coherent and spectrally incoherent excitation conditions. We speculate that the significant distinction between excitation conditions is not the coherence of light but rather the four-wave mixing signal itself. The nonlinear response—measured using coherent or incoherent light—allows measurements of dynamics that are hidden by averaging in experiments that use steady-state signals and theories that model the linear response of light-harvesting complexes illuminated by sunlight. Thus, the key challenge is to understand how four-wave mixing signals can reveal variables that are often hidden by averaging over time and ensembles. In Supplementary Note 4 and Supplementary Figs S11–S15 , we include preliminary measurements as a function of the waiting time, τ . In future work, we will further examine those results. The results demonstrate that I (4) 2D ES contains much the same as well as complementary information as femtosecond 2D ES. The measurements confirm the prediction [40] that it is possible to create, correlate and measure coherent superpositions during multiple time periods—in the present work coherences oscillating at optical frequencies as a function of interferometric delays σ and ζ —using incoherent excitation light. The results show that I (4) 2D ES is a sensitive probe of intermediates such as photoisomers that have long lifetimes and that coherent 2D optical spectroscopy measurements do not require femtosecond-pulse excitation. Experimental methods The measurement apparatus for time-integrated detection consisted of the light source described below, the same four-beam interferometer that was used previously [32] , [41] , and the detection scheme detailed below. Noisy-light measurements require a light source that is spectrally incoherent, broadband and bright enough to generate nonlinear optical signals. For technical convenience, spatial coherence is also desirable. Few currently available sources simultaneously satisfy those requirements. We used the ASE from the optical cavity of an unseeded Ti:sapphire amplifier pumped by a frequency-doubled yttrium lithium fluoride laser. The thermal cavity produced pulses with duration of about 150 ns, a repetition rate of 5 KHz and satisfactory spatial coherence. We measured the ASE pulse duration using a 1-ns-rise-time photodiode; Supplementary Fig. S6 displays an example trace. Without modification, the biggest drawbacks to this light source are the lack of tunability away from 800 nm and the relatively narrow bandwidth of about 30 nm. We addressed the second drawback by inserting a spectral shaping filter (Alpine Research Optics SF6040) into the optical cavity to reduce gain narrowing; the ASE bandwidth more than tripled to about 100 nm as shown in Fig. 2a . The bandwidth corresponds to a coherence time of about 20 fs. The total output power was about 200 mW. This beam was sent into the interferometer set-up where a 2D cross-hatched phase mask produced four copies in the standard square (BOX) formation. Ultraviolet-fused silica wedge pairs inserted into three beams correspond to interferometric delays σ , τ and ζ , where E A ( t ), E B ( t , σ), E C ( t , σ, τ) and E LO ( t , σ, τ, ζ). The interferometric delay variables ( σ , τ , ζ ) are analogous to the two common conventions in femtosecond 2D ES literature, ( τ 1 , τ 2 , τ 3 ) and ( τ , T , t ). Different words have also been used to describe each time interval. The first interval has been called the coherence or excitation time, the second is the waiting or population time and the third is the emission or signal or detection time. Each input beam was about 600 nJ per pulse before the sample without attenuation. This was well above the threshold needed to measure the phase-matched homodyne third-order signal in the direction. The beam waist radius at the focus was ~75 μm. Time-integrated detection involved a photodiode, a current preamplifier and data acquisition hardware for a personal computer. This equipment recorded a voltage value linearly related to the intensity of the heterodyned third-order nonlinear optical signal. One excitation beam was chopped at 500 Hz; the difference between the blocked and unblocked signals isolated the heterodyne signal, , from the homodyne contributions, and I LO . There was minimal residual scatter. Unsubtracted fluorescence from the excitation beam that was chopped led to the small non-zero background in the time-integrated data set shown in Fig. 1f . This non-zero background does not oscillate as a function of the interferometric delays and so it does not mar the I (4) 2D ES. Frequency-resolved detection involved a spectrometer and CCD, and one beam was chopped at 50 Hz. This detection set-up was constructed previously [41] and optimized for the visible spectrum. The throughput of the set-up from signal generation in the sample cell to detection at the CCD surface is >50% efficient at visible wavelengths. At 800 nm, the total efficiency of the same optics was <25%. At ~5 nJ per pulse, the electrical noise of the CCD was the largest source of noise. An optical apparatus optimized for 800 nm would increase efficiency significantly and would lead to detectable signals at excitation energies lower than 5 nJ per pulse. We used the DTP (Exciton), IR144 (Exciton) and solvents (Sigma-Aldrich) without further purification. Solvation of DTP in butanol red-shifted the absorption bands to improve the overlap of the sample and ASE spectra. The peak optical density in the 1-mm path length sample cell was <0.3. A gear pump flowed the sample at 150 ml min −1 in the time-integrated measurement and at 10 ml min −1 in the frequency-domain measurements to eliminate deleterious heating of the sample. The measurements were performed at room temperature. At ~5 nJ per pulse, the diffraction efficiency was about 0.004% for either DTP or IR144, which is on par with femtosecond experiments. It is productive to describe the magnitude of the signal and the scaling to other samples from the standpoint of kinetics; using light that is ‘always on’, chromophores will be excited and then either produce signal or de-excite via another channel such as fluorescence or photoisomerization. These processes are ongoing at all times. The steady-state terms describe signals whereby the two excitation beams excite a fraction of the molecules, and the third beam scatters from this equilibrium transient grating. To address the scaling of the steady-state contribution to the signal in a simplified manner, we consider a simple rate equation model for a two-level system; see for example, equation (7.4.6) in ref. 57 . We find that the steady-state density of molecules in the excited state, N , scales as , where A is the absorption cross-section of the sample, B is the excited-state lifetime and I is the laser intensity. The transient grating written into the sample will have an absorption modulation depth scaling as , and the grating efficiency will scale as . In the heterodyne-detected case, the steady-state terms scale as (see for example, equation (48) in ref. 40 ). Theoretical methods To build intuition about the I (4) 2D ES measurement, we describe linear absorption spectroscopy of a two-level system (|g and |e ) performed using a Michelson interferometer with quasi-cw incoherent excitation, as depicted in Fig. 1a–c . Linear absorption by a two-level system can be described by the first-order response function , where contains the frequency ( ) and assumes exponential dephasing ( ). Times t 1 and t 2 correspond to the excitation and emission field–matter interactions, respectively. The goal is to measure . The semiclassical initial field is , where is a complex stochastic function representing the random envelope and is the optical carrier frequency. Field interacts with the sample at time t 1 to produce a polarization that radiates an electric field, E sig , at a later time t 2 . We must account for all possible interaction times. Mathematically, this is given by . Without a sample, E— the field entering the interferometer—is . When a sample is inserted, E contains two components, , where for convenience we assume . Field E is split into two parts, fields and . The time-integrated signal at the photodiode is The signal of interest will be contained in the cross term ( I X ) Without a sample, the result is where the integral over t is a correlation function that simplifies to , assuming a light source of infinite bandwidth and of any spectral phase profile. The time-correlation function is depicted in Fig. 1b as brackets surrounding two wiggly lines representing the stochastic field envelopes. The result in equation (3) means that if the bandwidth were finite, oscillations at the carrier frequency would occur for a duration known as the coherence time. When a sample is present, the cross-term intensity becomes The signal from reproduces the temporal coherence profile of the excitation light (identical to equation (3)) and can be removed by a secondary measurement. The signal from leads to an oscillatory component containing the desired information, but this term is neglected in the low-density limit. The remaining terms from the expansion of equation (4) are the cross terms, which yield Insertion results in which can be simplified by the substitution and rearranged to yield and then solved with the conjugate term to produce the signal expression Incoherent excitation can indeed create coherent superpositions and allow measurement of dynamics much shorter than the pulse duration. In this case, the coherent superposition is between the ground and excited states, the dynamics are the optical dephasing and the pulse duration is cw. These oscillations are shown in Fig. 1c . Related descriptions of linear absorption can be found [58] , and similar concepts regarding coherence are exploited in other methods such as white-light interferometry and optical coherence tomography [59] . We have used linear absorption to illustrate an important general principle: measuring coherent oscillations and dynamics using an interferometer does not always require pulses with short temporal envelopes. In femtosecond 2D ES, it is customary to extract E sig at the field level [5] , [6] , [7] , [8] , [9] , [10] , [11] , [12] , [13] , [14] , [15] , [16] , [17] , [18] , [19] , [20] , [21] , [22] , [23] , [24] , [25] , [26] , [27] , [28] , [29] , [30] , [31] , [32] , [33] , [34] . In the example above, however, E sig at the field level is not very useful because it is a stochastic function of time. We are able to extract meaningful information about the sample, in this case , only by interferometric correlation. In I (4) 2D ES, a similar situation exists: E sig is a stochastic function of time and information can be obtained only by interferometric correlation. Therefore, linear absorption spectroscopy is a helpful basis for understanding I (4) 2D ES. The I (4) 2D ES theoretical analysis for time-integrated detection was detailed previously for a Bloch four-level system [40] and is outlined below. The analysis requires four fields and a large set of nonlinear response functions developed over three time periods between the field–matter interactions, . The key segment of the experimental apparatus is depicted in Fig. 1d . The measured intensity-level signals involve four-point time-correlation functions, which, under the standard assumption of circular complex Gaussian statistics, factorize into pairs of products of two-point correlation functions, . The factorization is depicted in Fig. 1e . An example starting expression—meaning the equivalent of equation (6)—is Examples of the final signal expressions are where is the lifetime of excited state |e 1 , and The first, equation (10), will lead to a diagonal peak at frequency coordinates , which does not depend on the value of τ , and the second example, equation (11), will lead to a cross peak at , which also does not depend on the value of τ . In these two example terms, the signal strength is related not only to the transition dipole moments, which is the same as femtosecond methods, but also to the excited-state lifetime. The third example, equation (12), will lead to a diagonal peak at that oscillates coherently as a function of τ at frequency , a quantum beat. The 128 expressions were categorized into three types based on the diagrammatic representation of the time-correlation functions: unrestricted, singly restricted and doubly restricted. Signals from the unrestricted terms, including the first and second examples above, were predicted to be strong because they fully integrate signal over the excited-state lifetime; such terms did not depend on τ . These signals are steady state, but they also contain information such as coupling or line broadening that is not directly measurable using linear spectroscopic methods. Signals from singly and doubly restricted terms do contain direct dynamics information during the waiting time τ , but they were expected to be weaker than signals because of unrestricted terms. This prediction depended on the ratio of the excited-state lifetime to the optical dephasing time. Finally, the method of coherent multidimensional spectroscopy using incoherent excitation was briefly used in NMR spectroscopy, and its history has been reviewed [60] . How to cite this article: Turner, D. B. et al. Coherent multidimensional optical spectra measured using incoherent light. Nat. Commun. 4:2298 doi: 10.1038/ncomms3298 (2013)